Wip1 deficiency impairs haematopoietic stem cell functionviap53 and mTORC1 pathways Wild-type p53-induced phosphatase 1 (Wip1) negatively regulates several tumour suppressor and DNA damage response pathways. However, the impact of Wip1 on haematopoietic stem cell (HSC) homeostasis and aging remains unknown. Here we show that Wip1 is highly expressed in HSCs but decreases with age. Wip1-deficient ( Wip1 −/− ) mice exhibited multifaceted HSC aging phenotypes, including the increased pool size and impaired repopulating activity. Deletion of p53 rescued the multilineage repopulation defect of Wip1 −/− HSCs without affecting cellular senescence or apoptosis, indicating that the Wip1–p53 axis regulates HSC differentiation in a manner independent of conventional p53 pathways. However, p53 deletion did not influence the increased HSC pool size in Wip1 −/− mice. Interestingly, the expansion of HSCs in Wip1 −/− mice was due to an mTORC1-mediated HSC proliferation. Thus, our study reveals a mechanism of stem cell aging, in which distinct effects of p53 and mTORC1 pathways on HSC aging are governed by Wip1. Haematopoietic stem cells (HSCs) reside at the top of the haematopoietic hierarchy and generate all types of haematopoietic progenitor cells (HPCs) and mature blood cells. The appropriate regulation of HSC function and maintenance is critical for the homeostasis of the haematopoietic system [1] . The regenerative capacity of HSCs declines with age [2] , [3] , [4] . However, the number of phenotypically defined HSCs in the bone marrow (BM) increases progressively with age in both mice and humans [3] , [4] , [5] , [6] , [7] . In addition, aged HSCs also exhibit a skewed differentiation potential towards generating decreased numbers of lymphoid cells but increased numbers of myeloid cells [2] , [6] , [8] , which are associated with impaired immune function and with increased incidence of myeloid leukaemia [3] , [7] , [9] , [10] . In connection to these observations, the proportion of myeloid-biased HSCs that are characterized by CD150 high and robust repopulating activity increases in the HSC population during aging. Meanwhile, the proportion of lymphoid-biased HSCs, which are characterized by CD150 low and moderate repopulating activity, decreases with age [7] , [11] . Tumour suppressor pathways have been implicated in maintaining haematopoietic homeostasis under both normal and stress conditions by regulating cell cycle, senescence and apoptosis in HSC compartments [12] , [13] , [14] , [15] , [16] , [17] . Wild-type (WT) p53-induced phosphatase 1 (Wip1 or PPM1D) negatively regulates the activity of multiple tumour suppression processes, including the p53, ATM, p16 (INK4a) and ARF pathways [18] , [19] . Recently, Wip1 has been implicated in the regulation of global heterochromatin silencing and, thus, is critical for maintaining genome integrity [20] . Wip1-deficient ( Wip1 −/− ) mice exhibit varied phenotypes including tumour resistance [21] , [22] , impaired adult neurogenesis [23] , [24] , obesity, atherosclerosis [25] and premature aging [26] , [27] . In the haematopoietic system, Wip1 deletion in mice results in a smaller thymus due to p53-dependent cell cycle arrest during the development of T cells [28] and enhanced maturation of neutrophils, which are mediated by p38 MAPK–STAT1-dependent pathways [29] . However, the role of Wip1 in regulating HSC homeostasis and aging remains unknown. In this study, we show that Wip1 −/− mice exhibit multiple aging-like phenotypes in HSCs, including a decline in their regenerative capacity and the phenotypic expansion of HSCs. Mechanistically, their impaired regenerative capacity is due to a p53-mediated differentiation defect in Wip1 −/− HSCs, whereas the increased number of Wip1 −/− HSCs is associated with the mammalian target of rapamycin complex 1 (mTORC1)-mediated cell cycle progression and proliferation of HSCs. Our findings provide a novel concept of HSC aging mediated by two distinct signalling pathways downstream of Wip1. Wip1 expression is high in HSCs and decreases with age Wip1 expression has been shown to decrease with age in pancreatic islets and in neural stem/progenitor cells [23] , [26] . To examine the expression levels of Wip1 mRNA in HSCs and HPCs, we purified long-term (LT) HSCs, short-term (ST) HSCs, multipotent progenitors and lineage-committed progenitors (common lymphoid progenitors; common myeloid progenitors; megakaryocyte-erythroid progenitors; and granulocyte–macrophage progenitors) from young (2- to 3-month-old) and old (20- to 24-month-old) WT mice via fluorescence-activated cell sorting (FACS), as depicted in Supplementary Fig. 1a . Among all of the analysed HSC and HPC subpopulations, the LT-HSCs displayed the highest expression level of Wip1 ( Fig. 1a ). Intriguingly, the Wip1 expression level in LT-HSCs progressively decreased with age ( Fig. 1b ). Western blot analysis showed that the Wip1 protein level was higher in lineage-negative BM cells than lineage-positive BM cells ( Supplementary Fig. 1b and 7f,g ) and decreased with age ( Supplementary Fig. 1c ), suggesting a potential role for Wip1 in regulating the aging process of HSCs. 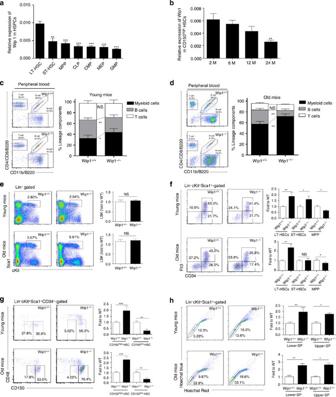Figure 1: Deletion of Wip1 leads to aging-like phenotypes in HSCs. (a)Wip1mRNA expression in LT-HSCs, ST-HSCs, multipotent progenitors (MPPs), common lymphoid progenitors (CLPs), common myeloid progenitors (CMPs), megakaryocyte-erythroid progenitors (MEPs) and granulocyte–macrophage progenitors (GMPs) from young (2-month-old) WT mice was measuredviareal-time PCR. The relative expression ofWip1was normalized to that of β-actin and compared with that in LT-HSCs for statistical analysis (n=5 mice). (b)Wip1mRNA expression in CD150high-HSCs from WT mice was measuredviareal-time PCR. The relative expression ofWip1was normalized to that of β-actin and compared with that in 2-month-old mice for statistical analysis (n=4 mice per group). M, month. (c,d) Representative FACS plots of myeloid (CD11b), B cells (B220) or T cells (CD4 and CD8). The bar graphs display the percentages of myeloid, B or T cells in PB in young mice (2- to 3-month-old;c) and in old (20- to 24-month-old) mice (d;n=5 mice per group). (e–h) Representative FACS plots of (e) LSK cells; (f) LT-HSCs, ST-HSCs and MPPs; (g) CD150high-HSCs and CD150low-HSCs; (h) lower-SP (side population) HSCs and upper-SP HSCs in young (2- to 3-month-old) and old (20- to 24-month-old) mice. The bar graphs display the relative number ofWip1−/−cells normalized to the average number ofWip1+/+(n=5 mice per group). All statistical data were assessed using Student’st-test and are presented as mean±s.d. *P<0.05; **P<0.01; ***P<0.001. NS, not significant. Figure 1: Deletion of Wip1 leads to aging-like phenotypes in HSCs. ( a ) Wip1 mRNA expression in LT-HSCs, ST-HSCs, multipotent progenitors (MPPs), common lymphoid progenitors (CLPs), common myeloid progenitors (CMPs), megakaryocyte-erythroid progenitors (MEPs) and granulocyte–macrophage progenitors (GMPs) from young (2-month-old) WT mice was measured via real-time PCR. The relative expression of Wip1 was normalized to that of β-actin and compared with that in LT-HSCs for statistical analysis ( n =5 mice). ( b ) Wip1 mRNA expression in CD150 high -HSCs from WT mice was measured via real-time PCR. The relative expression of Wip1 was normalized to that of β-actin and compared with that in 2-month-old mice for statistical analysis ( n =4 mice per group). M, month. ( c , d ) Representative FACS plots of myeloid (CD11b), B cells (B220) or T cells (CD4 and CD8). The bar graphs display the percentages of myeloid, B or T cells in PB in young mice (2- to 3-month-old; c ) and in old (20- to 24-month-old) mice ( d ; n =5 mice per group). ( e – h ) Representative FACS plots of ( e ) LSK cells; ( f ) LT-HSCs, ST-HSCs and MPPs; ( g ) CD150 high -HSCs and CD150 low -HSCs; ( h ) lower-SP (side population) HSCs and upper-SP HSCs in young (2- to 3-month-old) and old (20- to 24-month-old) mice. The bar graphs display the relative number of Wip1 −/− cells normalized to the average number of Wip1 +/+ ( n =5 mice per group). All statistical data were assessed using Student’s t -test and are presented as mean±s.d. * P <0.05; ** P <0.01; *** P <0.001. NS, not significant. Full size image Wip1 deletion results in age-associated phenotypes in HSCs To examine the effect of Wip1 deletion on the maintenance of haematopoiesis during aging, we analysed the peripheral blood (PB) in young and old Wip1 −/− mice. The Wip1 −/− mice exhibited a significant decrease in lymphoid cells and increase in myeloid cells in the PB of both young and old mice, indicating that Wip1 deletion induces haematopoietic differentiation skewing ( Fig. 1c,d ). No significant difference in the number of Lineage − Sca1 + c-Kit + (LSK) cells in BM was found ( Fig. 1e ); however, remarkable increases in the number of LT-HSCs in Wip1 −/− mice were detected at both young and old ages ( Fig. 1f ). To substantiate this finding, we performed additional flow cytometry-based experiments for further classification of the LT-HSCs ( Supplementary Fig. 1a ). In the CD34 − LSK cell population, the number of CD150 high CD48 – cells (CD150 high -HSCs) was dramatically increased, whereas the number of CD150 low CD48 − cells (CD150 low -HSCs) was depleted in Wip1 −/− mice ( Fig. 1g ). The LSK cell population in Wip1 −/− mice displayed a significant increase in both the upper and lower side populations ( Fig. 1h ). These data indicate that Wip1 deletion results in the haematopoietic differentiation skewing and the phenotypic expansion of HSCs, particularly in the most primitive HSCs. Deletion of Wip1 impairs the function of HSCs Because old HSCs tend to display decreased regenerative capacity after haematopoietic injury, we examined whether Wip1 deletion impairs the regeneration of HSCs after exposure to high-dose irradiation (IR) or 5-Fluoruracil (5-FU) treatment. Given that Wip1 deficiency also causes defects in nonhaematopoietic tissues, which might influence the survival time, we first transplanted Wip1 +/+ or Wip1 −/− BM cells into lethally irradiated WT recipient mice, and at 20 weeks post-transplantation, the recipient mice were exposed to 8 Gy IR or treated with 5-FU ( Supplementary Fig. 2a ). After IR or 5-FU treatment, the recipient mice reconstituted with Wip1 −/− BM cells died much faster than the recipient mice reconstituted with Wip1 +/+ BM cells ( Supplementary Fig. 2b,c ). To confirm the above findings, we performed competitive transplantation experiments and exposed the recipient mice to 4.5 Gy IR or 5-FU treatment at 16 weeks post-transplantation ( Supplementary Fig. 2d ). In contrast to that of the Wip1 +/+ controls, the percentage of donor-derived Wip1 −/− PB cells progressively decreased following 4.5 Gy IR or 5-FU treatment ( Supplementary Fig. 2e,f ). These data suggest that deletion of Wip1 in HSCs results in a functional defect. Next, we performed in vitro colony-forming assays. On the basis of the methylcellulose-based colony-forming unit (CFU) assay, the numbers of multipotent (CFU-Mix), erythroid (BFU-E) and myeloid (CFU-GM) progenitor cells in the total BM cells were comparable between the Wip1 +/+ and Wip1 −/− mice ( Fig. 2a ). However, the single-cell colony-forming ability of both the LT- and ST-HSCs was significantly reduced in the Wip1 −/− mice after 14 days of culturing in liquid medium containing cytokines ( Fig. 2b ). In the CD34 − LSK population, both the CD150 high and CD150 low cells from the Wip1 −/− mice displayed dramatic reductions in their single-cell colony-forming ability ( Fig. 2c ). 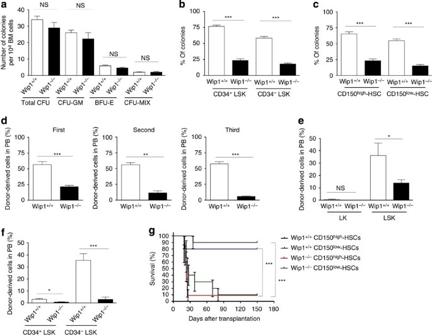Figure 2: Deletion ofWip1impairs the function of HSCs. (a) The number of progenitor cell colonies. In total, 1 × 104BM cells were cultured in methylcellulose medium for 14 days (n=4 mice per group). (b,c) Colonies were defined as consisting of more than 1,000 cells. Individual cell was sorted and cultured for 14 days in 96-well plates (n=5 mice per group). (d) The percentage of donor-derived PB cells at 20 weeks after serial transplantation. In total, 1 × 106BM cells were mixed with 1 × 106competitor BM cells for the first competitive transplantation. Overall, 5 × 106BM cells were serially transplanted for the second and third transplantations (n=5 mice per group). (e,f) The percentage of donor-derived PB cells at 20 weeks after transplantation. In total, 40,000 LK cells, 4,000 LSK cells, 100 CD34+LSK cells or 100 CD34−LSK cells were mixed with 5 × 105competitor BM cells for competitive transplantation (n=5 mice per group). (g) Survival curves of the recipient mice transplanted with 50 CD150high-HSCs or 50 CD150low-HSCs mixed with 3 × 105Sca1−BM cells (n=10 per group). All statistical data were assessed using Student’st-test and are presented as mean±s.d. *P<0.05; **P<0.01; ***P<0.001. NS, not significant. Figure 2: Deletion of Wip1 impairs the function of HSCs. ( a ) The number of progenitor cell colonies. In total, 1 × 10 4 BM cells were cultured in methylcellulose medium for 14 days ( n =4 mice per group). ( b , c ) Colonies were defined as consisting of more than 1,000 cells. Individual cell was sorted and cultured for 14 days in 96-well plates ( n =5 mice per group). ( d ) The percentage of donor-derived PB cells at 20 weeks after serial transplantation. In total, 1 × 10 6 BM cells were mixed with 1 × 10 6 competitor BM cells for the first competitive transplantation. Overall, 5 × 10 6 BM cells were serially transplanted for the second and third transplantations ( n =5 mice per group). ( e , f ) The percentage of donor-derived PB cells at 20 weeks after transplantation. In total, 40,000 LK cells, 4,000 LSK cells, 100 CD34 + LSK cells or 100 CD34 − LSK cells were mixed with 5 × 10 5 competitor BM cells for competitive transplantation ( n =5 mice per group). ( g ) Survival curves of the recipient mice transplanted with 50 CD150 high -HSCs or 50 CD150 low -HSCs mixed with 3 × 10 5 Sca1 − BM cells ( n =10 per group). All statistical data were assessed using Student’s t -test and are presented as mean±s.d. * P <0.05; ** P <0.01; *** P <0.001. NS, not significant. Full size image To examine the in vivo function of Wip1 −/− HSCs, we performed competitive BM transplantation experiments. The percentage of Wip1 −/− donor-derived PB cells was significantly lower in the primary transplant and progressively declined in the serial transplants ( Fig. 2d ). To verify this result, we performed competitive transplantation experiments using Lineage − c-Kit + Sca1 − (LK), LSK, CD34 + LSK and CD34 − LSK cells. Neither the Wip1 −/− nor the Wip1 +/+ LK cells showed long-term multilineage reconstitution, whereas the Wip1 −/− LSK cells displayed significantly reduced regenerative capacity compared with the Wip1 +/+ LSK cells ( Fig. 2e ). Interestingly, the CD34 − LSK cells displayed a greater defect than the CD34 + LSK cells ( Fig. 2f ), suggesting a specific role of Wip1 in the most primitive HSCs. Furthermore, we co-transplanted 50 purified CD150 high -HSCs or CD150 low -HSCs with HSC-depleted competitor cells (3 × 10 5 Sca1 − BM cells) into lethally irradiated mice. Most of the recipient mice transplanted with the Wip1 −/− CD150 high -HSCs or CD150 low -HSCs died within 4 weeks, whereas most of the recipient mice transplanted with the Wip1 +/+ CD150 high -HSCs or CD150 low -HSCs survived for at least 150 days ( Fig. 2g ). These data demonstrate that Wip1 deletion leads to a profound failure of HSCs to generate colonies in vitro and to reconstitute haematopoietic system of lethally irradiated mice. Wip1 deficiency induces HSC cell-intrinsic defects The above data indicate that Wip1 deletion in mice results in aging-like phenotypes in HSCs, including increased number, skewed haematopoietic differentiation and impaired repopulation capacity of HSCs. To determine whether these changes are due to cell-intrinsic or cell-extrinsic mechanisms, we performed uncompetitive transplantation ( Supplementary Fig. 3a ) and reciprocal BM transplantation ( Supplementary Fig. 3e ) experiments and killed the recipient mice for FACS analysis and single-cell colony-forming assay 20 weeks post-transplantation. The phenotypes of skewed differentiation and expanded HSCs were only detected in the Wip1 −/− donor-derived BM cells but not in the Wip1 +/+ donor-derived BM cells regardless of the genotype of the recipient mice ( Supplementary Fig. 3b,c,f,g ). The Wip1 −/− donor-derived HSCs displayed a remarkably reduced single-cell colony-forming capacity compared with the Wip1 +/+ donor-derived HSCs regardless of the host genotypes ( Supplementary Fig. 3d,h ). These data indicate that Wip1 deficiency induces aging-like phenotypes in HSCs via cell-autonomous mechanisms. Deletion of Wip1 results in a defect in HSC differentiation The aging-like phenotypes of Wip1 −/− HSCs prompted us to examine the markers of cellular senescence and apoptosis in Wip1 −/− HSCs. However, we did not detect any difference in the senescence-associated β-gal activity ( Supplementary Fig. 4a ), the expression levels of p16 ( Supplementary Fig. 4b ) or the Annexin V-positive cells between the Wip1 −/− and Wip1 +/+ HSCs ( Supplementary Fig. 4c ), indicating that the impaired regenerative capacity of HSCs is not due to cellular senescence or apoptosis. A recent study demonstrated that the proportion of old-donor-derived HSCs in the BM is substantially higher than that predicted based on the proportion of old-donor-derived cells in the PB in competitive transplantation experiment, indicating a decreased differentiating activity in aged HSCs [30] . To examine whether the impaired repopulating capacity of Wip1 −/− HSCs is due to a defect in their differentiation capacity, we examined the percentage of donor-derived cells in HSC and HPC subpopulations in BM cells from primary, secondary and tertiary recipient mice at 20 weeks post-transplantation. Interestingly, the percentage of donor-derived Wip1 −/− cells in the CD34 − LSK cells in the primary recipient mice is comparable to that of the Wip1 +/+ controls; however, the percentage of donor-derived Wip1 −/− cells in the CD34 + LSK cells was significantly reduced, and a further reduction was detected in more differentiated HPCs ( Fig. 3a ), indicating a continuous impairment in differentiation capacity at multiple steps. In the secondary and tertiary transplantations, the percentage of donor-derived Wip1 −/− cells displayed a relative increase in the CD34 − LSK cell compartment but a further decrease in the CD34 + LSK cell compartment ( Fig. 3b,c ), suggesting that serial transplantation might accelerate the HSC expansion and exacerbate the HSC differentiation defect induced by Wip1 deficiency. Similar results were found on the basis of competitive LSK cell transplantation experiments ( Fig. 3d ). In addition, the Wip1 −/− mice exhibited a significant depletion of CD150 low -HSCs ( Fig. 1g ), whereas the cell cycle status and apoptosis rate of the CD150 low -HSCs were comparable between the Wip1 −/− and Wip1 +/+ mice ( Supplementary Fig. 4d,e ), suggesting that the differentiation capacity of CD150 high -HSCs into CD150 low -HSCs is impaired in Wip1 −/− mice. These data indicate that Wip1 deficiency impairs HSC differentiation at multiple steps but particularly the early stage of differentiation, which results in repopulation defect of HSCs in Wip1 −/− mice. 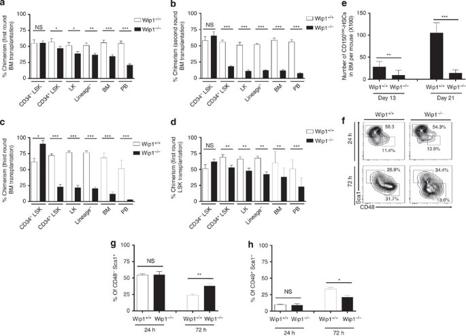Figure 3: Deletion ofWip1results in a defect in HSC differentiation. (a–c) The percentage of donor-derived BM or PB cells at 20 weeks after transplantation. In total, 1 × 106BM cells were mixed with 1 × 106competitor cells for the first competitive transplantation (a). In total, 5 × 106BM cells were serially transplanted for the second (b) and third (c) transplantations (n=5–8 mice per group). (d) The percentage of donor-derived BM or PB cells at 20 weeks after transplantation. In total, 4,000 LSK cells were mixed with 5 × 105competitor BM cells for competitive transplantation (n=8 per group). (e) The number of CD150low-HSCs in BM per mouse at the indicated time point after 5-FU treatment (n=5 per group). (f) Representative FACS plots of stem cells (CD48−Sca1+) and progenitor cells (CD48+Sca1−) in culture. (g) The percentage of undifferentiated haematopoietic cells (CD48−Sca1+) in culture (n=5 mice per group). (h) The percentage of differentiated haematopoietic cells (CD48+Sca1−) in culture (n=5 mice per group). All statistical data were assessed using Student’st-test and are presented as mean±s.d. *P<0.05; **P<0.01; ***P<0.001. NS, not significant. Figure 3: Deletion of Wip1 results in a defect in HSC differentiation. ( a – c ) The percentage of donor-derived BM or PB cells at 20 weeks after transplantation. In total, 1 × 10 6 BM cells were mixed with 1 × 10 6 competitor cells for the first competitive transplantation ( a ). In total, 5 × 10 6 BM cells were serially transplanted for the second ( b ) and third ( c ) transplantations ( n =5–8 mice per group). ( d ) The percentage of donor-derived BM or PB cells at 20 weeks after transplantation. In total, 4,000 LSK cells were mixed with 5 × 10 5 competitor BM cells for competitive transplantation ( n =8 per group). ( e ) The number of CD150 low -HSCs in BM per mouse at the indicated time point after 5-FU treatment ( n =5 per group). ( f ) Representative FACS plots of stem cells (CD48 − Sca1 + ) and progenitor cells (CD48 + Sca1 − ) in culture. ( g ) The percentage of undifferentiated haematopoietic cells (CD48 − Sca1 + ) in culture ( n =5 mice per group). ( h ) The percentage of differentiated haematopoietic cells (CD48 + Sca1 − ) in culture ( n =5 mice per group). All statistical data were assessed using Student’s t -test and are presented as mean±s.d. * P <0.05; ** P <0.01; *** P <0.001. NS, not significant. Full size image To further investigate the differentiation defect of HSCs in Wip1 −/− mice, we treated mice with 5-FU and analysed the recovery of CD150 low -HSCs via FACS. Wip1 −/− mice shown less CD150 low -HSCs in the spleen compared with Wip1 +/+ mice ( Supplementary Fig. 4f ). More obviously, the recovery of CD150 low -HSCs in the BM was significantly impaired in the Wip1 −/− mice compared with the Wip1 +/+ mice ( Fig. 3e ). Ki67 and Annexin V staining did not indicate any difference in cell proliferation or apoptosis, respectively, between the Wip1 −/− and Wip1 +/+ CD150 low -HSCs ( Supplementary Fig. 4g,h ). Furthermore, we examined the differentiation defect of Wip1 −/− CD150 high -HSCs in culture. Wip1 −/− cultures displayed a significantly higher proportion of undifferentiated cells (Lineage − CD48 − Sca1 + ) and a significantly lower proportion of differentiated cells (Lineage − CD48 + Sca1 − ; Fig. 3f–h ). Again, no difference in the rate of cell proliferation or apoptosis was detected in the Wip1 −/− and Wip1 +/+ cultures ( Supplementary Fig. 4i,j ). These data reinforced the notion that Wip1 deficiency results in decreased HSC differentiation capacity. Wip1 −/− HSCs show increased proliferation The phenotypic expansion of HSCs is another important characteristic of old HSCs that is recapitulated in Wip1 −/− mice ( Fig. 1f–h ). To understand the mechanism underlying the phenotypic expansion of HSCs in Wip1 −/− mice, we examined 5-bromodeoxyuridine (BrdU) incorporation of BM cells in 10-day BrdU-labelled mice. Interestingly, both the LSK cells and the CD34 − LSK cells from the Wip1 −/− mice displayed a moderate but significant increase in their long-term proliferation rate ( Fig. 4a,b ). Next, we treated the mice with 5-FU or PIPC, and found that significantly more Wip1 −/− HSCs enter the cell cycle than Wip1 +/+ HSCs on proliferative stimulations ( Fig. 4c,d ). Thus, these data suggest that Wip1 deficiency induces HSC proliferation, which may contribute to the phenotypic expansion of the Wip1 −/− HSCs. 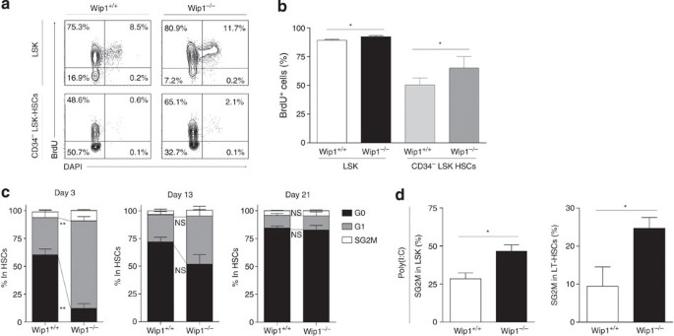Figure 4:Wip1−/−HSCs show increased proliferation. (a) Representative FACS plots of BrdU staining of LSK cells and CD34−Flt3−LSK cells after 10 days of BrdU labelling. (b) Bar graph displays the percentage of BrdU-positive cells in LSK and CD34−Flt3−LSK as indicated (n=4 mice per group). (c) The cell cycle profiles of the CD150high-HSCs were determined by Ki67 staining at the indicated time point after 5-FU treatment (n=5 mice per group). (d) The percentages of cells in the S and G2/M phases in the LSK cells and LT-HSCs cells were determined by Ki67 staining 2 days after the PIPC treatment (n=5 mice per group). All statistical data were assessed using Student’st-test and are presented as mean±s.d. *P<0.05; **P<0.01. NS, not significant. Figure 4: Wip1 −/− HSCs show increased proliferation. ( a ) Representative FACS plots of BrdU staining of LSK cells and CD34 − Flt3 − LSK cells after 10 days of BrdU labelling. ( b ) Bar graph displays the percentage of BrdU-positive cells in LSK and CD34 − Flt3 − LSK as indicated ( n =4 mice per group). ( c ) The cell cycle profiles of the CD150 high -HSCs were determined by Ki67 staining at the indicated time point after 5-FU treatment ( n =5 mice per group). ( d ) The percentages of cells in the S and G2/M phases in the LSK cells and LT-HSCs cells were determined by Ki67 staining 2 days after the PIPC treatment ( n =5 mice per group). All statistical data were assessed using Student’s t -test and are presented as mean±s.d. * P <0.05; ** P <0.01. NS, not significant. Full size image Impaired function of Wip1 −/− HSCs is due to p53 activation Previous studies have shown that Wip1 deficiency results in sustained p53 activation, which impairs the function of neural and intestinal stem cells via cell cycle arrest and apoptosis, respectively [21] , [24] . Although the Wip1 −/− HSCs did not display any increase in cell cycle arrest or apoptosis, we did detect significant upregulation of p53 downstream target genes in Wip1 −/− HSCs after transplantation ( Fig. 5a ). Western blot analysis confirmed p53 activation in the Wip1 −/− HSCs, as indicated by a significant increase in the level of phosphorylated p53 ( Fig. 5b and Supplementary Fig. 7a–c ). 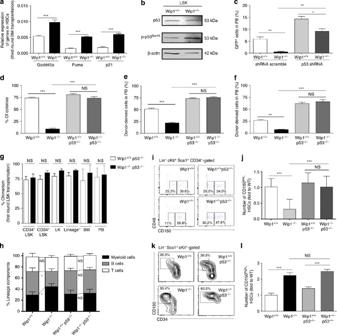Figure 5: TheWip1–p53 axis impairs HSC differentiation. (a) Relative expression levels of Gadd45a, Puma and p21 were normalized to that of β-actin in CD150high-HSCs after BM transplantation (n=5 mice per group). (b) Representative western blots show p53 and p-p53Ser15expression in freshly isolated LSK cells (n=5 mice per group were pooled). (c) The percentage of GFP+cells in the PB at 20 weeks after transplantation. The LSK cells were infected with p53-shRNA or scramble-shRNA lentivirus, and the transduced cells (GFP+) were sorted for the competitive repopulating assay (n=5 mice per group). (d) The percentage of colonies consisting of more than 1,000 cells. Single-cell colony-forming assay was performed on sorted individual CD150high-HSC (n=4 mice per group). (e) The percentage of donor-derived PB cells at 20 weeks after transplantation. In total, 1 × 106BM cells were used for the primary competitive transplantation (n=5 mice per group). (f) The percentage of donor-derived PB cells at 20 weeks after transplantation. In total, 4,000 LSK cells were used for competitive transplantation (n=5 mice per group). (g) The percentage of donor-derived BM or PB cells at 20 weeks after transplantation. In total, 4,000 LSK cells were mixed with 5 × 105competitor BM cells for competitive transplantation (n=5 per group). (h) The bars show percentages of the cells that expressed myeloid (CD11b), B cell (B220) or T cell (CD4 and CD8) lineage markers in PB (n=5 per group). (i) Representative FACS plots of CD150high-HSCs and CD150low-HSCs. (j) The relative number of CD150low-HSCs normalized to the average number ofWip1+/+(n=5 mice per group). (k) Representative FACS plots display the percentage of CD150highcells in the LSK cells. (l) The relative number of CD150high-HSCs normalized to the average number ofWip1+/+(n=5 mice per group). All statistical data were assessed using Student’st-test and are presented as mean±s.d. *P<0.05; **P<0.01; ***P<0.001. NS, not significant. Figure 5: The Wip1 –p53 axis impairs HSC differentiation. ( a ) Relative expression levels of Gadd45a, Puma and p21 were normalized to that of β-actin in CD150 high -HSCs after BM transplantation ( n =5 mice per group). ( b ) Representative western blots show p53 and p-p53 Ser15 expression in freshly isolated LSK cells ( n =5 mice per group were pooled). ( c ) The percentage of GFP + cells in the PB at 20 weeks after transplantation. The LSK cells were infected with p53-shRNA or scramble-shRNA lentivirus, and the transduced cells (GFP + ) were sorted for the competitive repopulating assay ( n =5 mice per group). ( d ) The percentage of colonies consisting of more than 1,000 cells. Single-cell colony-forming assay was performed on sorted individual CD150 high -HSC ( n =4 mice per group). ( e ) The percentage of donor-derived PB cells at 20 weeks after transplantation. In total, 1 × 10 6 BM cells were used for the primary competitive transplantation ( n =5 mice per group). ( f ) The percentage of donor-derived PB cells at 20 weeks after transplantation. In total, 4,000 LSK cells were used for competitive transplantation ( n =5 mice per group). ( g ) The percentage of donor-derived BM or PB cells at 20 weeks after transplantation. In total, 4,000 LSK cells were mixed with 5 × 10 5 competitor BM cells for competitive transplantation ( n =5 per group). ( h ) The bars show percentages of the cells that expressed myeloid (CD11b), B cell (B220) or T cell (CD4 and CD8) lineage markers in PB ( n =5 per group). ( i ) Representative FACS plots of CD150 high -HSCs and CD150 low -HSCs. ( j ) The relative number of CD150 low -HSCs normalized to the average number of Wip1 +/+ ( n =5 mice per group). ( k ) Representative FACS plots display the percentage of CD150 high cells in the LSK cells. ( l ) The relative number of CD150 high -HSCs normalized to the average number of Wip1 +/+ ( n =5 mice per group). All statistical data were assessed using Student’s t -test and are presented as mean±s.d. * P <0.05; ** P <0.01; *** P <0.001. NS, not significant. Full size image To determine the potential role of p53 in mediating the functional defect in Wip1 −/− HSCs, we performed a knockdown experiment using a lentivirus-mediated short hairpin RNA (shRNA) targeting p53. Transduced LSK cells were subjected to a competitive transplantation experiment ( Supplementary Fig. 5a ). Knockdown of p53 significantly improved the regenerative capacity of the Wip1 −/− HSCs ( Fig. 5c ). To verify this result, we generated Wip1 −/− p53 −/− double-mutant mice and performed in vitro and in vivo functional assays. The single-cell colony-forming assay revealed a significant improvement in the in vitro function of the Wip1 −/− p53 −/− HSCs ( Fig. 5d ). Competitive BM transplantation experiments revealed a complete rescue of the regenerative defect in the Wip1 −/− p53 −/− HSCs ( Fig. 5e ), and this rescue was sustained in secondary BM transplants ( Supplementary Fig. 5b ). Similar data were obtained from competitive HSC transplantation experiments, demonstrating that p53 deletion completely rescued the repopulation defect of Wip1 −/− HSCs ( Fig. 5f ). To determine whether p53 deletion rescued the repopulation capacity of Wip1 −/− HSCs by ameliorating the HSC differentiation defect, we analysed the percentage of donor-derived cells in HSC and HPC subpopulations of the primary recipient mice. The results revealed that p53 deletion significantly ameliorated the HSC differentiation defect in the Wip1 −/− HSCs at multiple steps ( Fig. 5g ). Furthermore, the skewed differentiation and the depletion of CD150 low -HSCs induced by Wip1 deficiency were completely rescued by p53 deletion ( Fig. 5h–j ). These data suggest that Wip1 deletion induces sustained p53 activation, leading to the HSC differentiation defect, thereby impairing the regenerative capacity of Wip1 −/− HSCs. Previous studies showed that modification of p53 expression or activity affects HSC self-renewal and number [31] , [32] . To determine whether the HSC expansion in Wip1 −/− mice is dependent on the p53 pathway, we examined the percentage of HSCs in Wip1 −/− p53 −/− mice. The proportion of CD150 high -HSCs remained significantly higher in Wip1 −/− p53 −/− mice ( Fig. 5k,l ). These data suggest that Wip1 deficiency induces the phenotypic expansion of HSCs via a p53-independent mechanism. One major transcriptional target of p53 is cyclin-dependent kinase inhibitor 1A (p21), which mediates G1 cell-cycle arrest in HSCs [33] . To examine whether p53-mediated differentiation defect in Wip1 −/− HSCs is dependent on p21, we generated Wip1 −/− p21 −/− double-mutant mice by crossing Wip1 +/− mice with p21 +/− mice. As expected, the Wip1 −/− p21 −/− mice showed increased number of HSCs similarly to Wip1 −/− p53 −/− or Wip1 −/− mice ( Supplementary Fig. 6a,b ). The defect in the single-cell colony-forming ability was not rescued in the Wip1 −/− p21 −/− HSCs ( Supplementary Fig. 6c ). On the basis of competitive repopulation assays using either total BM cells or FACS-sorted HSCs, the Wip1 −/− p21 −/− HSCs did not display any improvement in their regenerative capacity compared with the Wip1 −/− p21 +/+ HSCs ( Supplementary Fig. 6d,e ). These results indicated that regulation of HSC differentiation by p53 is independent of p21. Because Wip1 also dephosphorylates many other proteins that have been implicated in the regulation of HSC function, such as p38 and NF-κB p65 (refs 34 , 35 ), we also determined the potential role of p38 and NF-κB in the function of Wip1 −/− HSCs via single-cell colony-forming assays. The results revealed that neither a p38 inhibitor nor a NF-κB inhibitor rescued the impaired function of the Wip1 −/− HSCs ( Supplementary Fig. 6f,g ). Phenotypic expansion of Wip1 −/− HSCs depends on mTORC1 We showed that the Wip1–p53 axis regulates HSC differentiation, but not HSC proliferation. To identify novel potential regulators of the phenotypic expansion of HSCs in Wip1 −/− mice, we performed global gene expression profiling ( Supplementary Table. 1 ). As expected, ingenuity pathway analysis (IPA) revealed an enrichment of differentially expressed genes related to the p53 pathway. In addition, this analysis also revealed a significant enrichment of differentially expressed genes related to protein synthesis and fatty acid metabolism, therefore predicting mTORC1 as a potential regulator of HSC phenotypic expansion ( Fig. 6a ). To verify this finding, we analysed the expression level of phospho-p70S6K (Thr389), an indicator of mTORC1 activity, via western blot analysis and found that Lineage − c-Kit + BM cells from Wip1 −/− mice displayed a significant increase in the level of phospho-p70S6K (Thr389) expression ( Fig. 6b and Supplementary Fig. 7d,e ). mTORC1 pathway activation has been associated with the HSC cycling in old HSCs [36] . Therefore, we speculated that the inhibition of Wip1 might induce the HSC proliferation, thereby increasing the number of HSCs via an mTORC1-dependent mechanism. 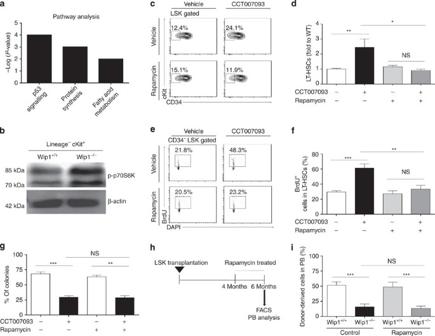Figure 6: Phenotypic expansion ofWip1−/−HSCs depends on mTORC1. (a) Microarray-based IPA of theWip1+/+andWip1−/−HSCs. The IPA results are expressed as –log (Pvalue). (b) Representative western blots show phosphorylated p70S6K expression in freshly isolated Lineage−c-Kit+BM cells (n=5 mice per group were pooled). (c) Representative FACS plots display the percentage of CD34−cells in the LSK cells from Wip1 inhibitor CCT007093- or rapamycin-treated WT mice. (d) The relative number of LT-HSCs normalized to the average number ofWip1+/+(n=5 mice per group). (e) Representative FACS plots show the percentage of BrdU-positive cells in the CD34−Flt3−LSK cells (LT-HSCs). (f) Bar graph shows the percentage of BrdU-positive cells in the LT-HSCs (n=5 mice per group). (g) Individual CD150high-HSC was sorted from WT mice treated with or without a Wip1 inhibitor (CCT007093) and/or an mTORC1 inhibitor (rapamycin). At 14 days after culture, the numbers of colonies consisting of more than 1,000 cells were counted (n=5 per group). (h) Schematic diagram of competitive transplantation and rapamycin treatment. In total, 4,000 LSK cells were mixed with 1 × 106competitor cells and transplanted. Four months later, the recipient mice were treated with rapamycin in drinking water for 2 months. (i) Percentage of donor-derived cells in the PB after the rapamycin treatment was determinedviaFACS analysis (n=5 mice per group). All statistical data were assessed using Student’st-test and are presented as mean±s.d. *P<0.05; **P<0.01; ***P<0.001. NS, not significant. Figure 6: Phenotypic expansion of Wip1 −/− HSCs depends on mTORC1. ( a ) Microarray-based IPA of the Wip1 +/+ and Wip1 −/− HSCs. The IPA results are expressed as –log ( P value). ( b ) Representative western blots show phosphorylated p70S6K expression in freshly isolated Lineage − c-Kit + BM cells ( n =5 mice per group were pooled). ( c ) Representative FACS plots display the percentage of CD34 − cells in the LSK cells from Wip1 inhibitor CCT007093- or rapamycin-treated WT mice. ( d ) The relative number of LT-HSCs normalized to the average number of Wip1 +/+ ( n =5 mice per group). ( e ) Representative FACS plots show the percentage of BrdU-positive cells in the CD34 − Flt3 − LSK cells (LT-HSCs). ( f ) Bar graph shows the percentage of BrdU-positive cells in the LT-HSCs ( n =5 mice per group). ( g ) Individual CD150 high -HSC was sorted from WT mice treated with or without a Wip1 inhibitor (CCT007093) and/or an mTORC1 inhibitor (rapamycin). At 14 days after culture, the numbers of colonies consisting of more than 1,000 cells were counted ( n =5 per group). ( h ) Schematic diagram of competitive transplantation and rapamycin treatment. In total, 4,000 LSK cells were mixed with 1 × 10 6 competitor cells and transplanted. Four months later, the recipient mice were treated with rapamycin in drinking water for 2 months. ( i ) Percentage of donor-derived cells in the PB after the rapamycin treatment was determined via FACS analysis ( n =5 mice per group). All statistical data were assessed using Student’s t -test and are presented as mean±s.d. * P <0.05; ** P <0.01; *** P <0.001. NS, not significant. Full size image To examine this hypothesis, we treated WT mice with the Wip1 inhibitor CCT007093 via intraperitoneal injection twice a day for 3 days. The Wip1 inhibitor-treated mice displayed a significant increase in the number of HSCs compared with the vehicle-treated controls ( Fig. 6c,d ). Interestingly, treatment with the mTORC1 inhibitor rapamycin completely blocked the Wip1 inhibitor-induced phenotypic expansion of HSCs ( Fig. 6c,d ). A BrdU incorporation assay revealed that the Wip1 inhibitor treatment significantly increased the proliferation rate of HSCs, which was completely blocked by rapamycin treatment ( Fig. 6e,f ). Next, we examined whether mTORC1 is involved in the regulation of HSC differentiation in Wip1 −/− mice. The HSCs from WT mice treated with the Wip1 inhibitor displayed significantly reduced single-cell colony-forming capacities; however, this reduction was not rescued by the rapamycin treatment ( Fig. 6g ). To substantiate this finding, we performed competitive transplantation experiments and treated the recipient mice with rapamycin ( Fig. 6h ). The results revealed that the rapamycin treatment did not affect the percentage of donor-derived Wip1 −/− PB cells, indicating that inhibiting mTORC1 does not improve the differentiation of Wip1 −/− HSCs ( Fig. 6i ). Taken together, these data indicate that Wip1 deletion results in sustained mTORC1 activation inducing the HSC cycling and thereby leading to the phenotypic expansion of HSCs, which is independent of the impaired differentiation capacity of Wip1 −/− HSCs. The balance between HSC self-renewal and differentiation is critical to sustain lifelong blood cell production. During aging, the progressive loss of this balance between self-renewal and differentiation is associated with decreased regenerative potential, increased HSC quantities and biased differentiation [3] , [4] , [5] , [8] . These aging phenotypes of HSCs are associated with age-related haematopoietic disorders, such as diminished immune function or increased myeloid leukaemia [7] , [10] , [14] . Although p53 and mTORC1 have been implicated in HSC aging, the mechanism by which these p53–mTORC1 interactions might play a role in cellular senescence and organismal aging remains unclear. In this study, we found that p53 and mTORC1 pathways, respectively, regulate two aging-like phenotypes in HSCs, that is, HSC functionality and phenotypic expansion, both of which are orchestrated by Wip1. Recent studies suggest that Wip1 plays an important role in regulating certain physiological and pathological processes by dephosphorylating distinct downstream targets [21] , [24] , [25] , [26] , [29] , [37] . In pancreatic islets, reduced Wip1 expression contributes to the aging-related decline in the proliferation and regenerative capacities of pancreatic islets via increased p38 activity [26] . In the subventricular zone, decreased Wip1 expression contributes to neuron formation defects via increased DKK3 activity, which inhibits the Wnt signalling pathway [23] . Our study showed that Wip1 expression progressively reduces with age in HSCs and Wip1 deletion accelerates HSC aging by increasing p53 and mTORC1 activities. Altered p53 activity has been implicated in HSC aging, affecting both HSC frequency and self-renewal [15] , [31] , [38] . Mutant mice carrying a hypermorphic p53 allele exhibit premature aging and impaired HSC self-renewal capacity [31] , [39] . However, ‘super-p53’ mice, which carry three copies of WT p53, exhibit no evidence of accelerated aging [40] . Therefore, the constitutively hyperactive p53 function accelerates aging in the p53 hypermorphic mice, whereas the expression of an extra copy of p53 under normal conditions does not accelerate aging in the ‘super-p53’ mice. In our study, Wip1 deletion resulted in a sustained moderate activation of p53 under physiological conditions, which promoted the aging process in HSCs. Interestingly, the impaired functionality of Wip1 −/− HSCs is not due to the well-known function of p53 in regulating cellular senescence, apoptosis, cell cycle or HSC self-renewal but rather the reduced differentiation capacity. Similarly, a recent study demonstrated that depleting PTPMT1, a PTEN-like mitochondrial phosphatase, results in haematopoietic failure due to the strong inhibition of HSC differentiation [41] . Another study demonstrated that conditionally ablating Dnmt3a, a DNA methyltransferase, leads to the progressive impairment of HSC differentiation over serial transplantations [42] . In addition, a recent study using bar-coding-based quantitative clonal analysis demonstrated that the proportion of old-donor-derived HSCs in the BM is substantially higher than that predicted according to the proportion of old-donor-derived PB cells on the basis of competitive transplantation experiments, indicating that old HSCs display compromised differentiation capacity [30] . Consistent with this finding, the increase in DNA methylation at transcription factor-binding sites that are associated with differentiation-promoting genes reinforces the diminished differentiation capacity in old HSC [43] . In agreement with these data, our results show that Wip1 deletion results in an impairment in HSC differentiation, particularly in the transition from most primitive HSCs to less primitive HSCs, which is completely rescued by p53 deletion. Altogether, these data revealed a novel function of p53 in regulating HSC differentiation, and suggested that dysregulation of the Wip1–p53 pathway induces HSC aging by reducing the differentiation capacity of HSCs. Previous studies using mouse models exhibiting telomere dysfunction-induced premature aging phenotypes demonstrated that p53 pathway activation impairs HSC maintenance and function with age [38] . A recent study of Fanconi anaemia patients showed that an overactive p53/p21 stress response and cell cycle arrest are responsible for the observed progressive HSC depletion and BM failure [44] . However, in our study, the impairment in HSC differentiation capacity appears to be independent of p21 upregulation. Consistent with our data, a previous study showed that the regulation of HSC quiescence and self-renewal by p53 did not involve p21 but rather was related to other p53 target genes [32] . In fact, our previous study demonstrated that p21 upregulation limits the function of HSCs with dysfunctional telomeres but not those with normal telomeres [38] . Therefore, p21 upregulation in response to p53 activation may regulate HSC aging, depending on the level of DNA damage and telomere function. The number of phenotypically defined HSCs increases with age in both humans and mice [4] , [5] , [6] , [7] ; however, the underlying mechanisms are largely unknown. In WT mice, mTORC1 activity increases in HSCs with age, and treatment with rapamycin reversed some of the aging phenotypes in old HSCs [45] . Consistently, our data showed that the rapamycin treatment abolished the phenotypic expansion of HSCs in Wip1 inhibitor-treated mice, implicating that mTORC1 activity is regulated by Wip1 in HSCs. A variety of genetic mouse models have shown that increased mTORC1 activity induces HSC hyperproliferation and a loss of quiescence, which ultimately leads to HSC exhaustion [36] , [46] , [47] , [48] . However, activation of mTORC1 by Wip1 deletion did not lead to HSC exhaustion in the transplantation experiments of Wip1 −/− or Wip1 −/− p53 −/− BM cells. Thus, moderate activation of mTORC1 induces HSC phenotypic expansion, whereas a drastic increase in mTORC1 activity depletes HSCs. Proper activation of mTORC1 may allow us to control HSC self-renewal and expansion of HSCs in vitro . In summary, our study provides a novel concept of HSC aging that two distinct pathways downstream of Wip1 contribute to two different HSC aging phenotypes. The findings suggest that controlling Wip1 may prevent the aging of HSCs. On the other hand, the potentially beneficial role of a Wip1 inhibitor in cancer treatment [49] might come at a cost of accelerated aging in HSC compartments. Given that Wip1 deficiency impairs HSC function via a p53-dependent but p21-independent differentiation checkpoint, determining the direct target of p53 that regulates the differentiation decision of HSCs will be of great interest. Because the p53 and mTORC1 pathways are responsible for these two aging-like phenotypes in HSCs, both of which are orchestrated by Wip1, exploring the potential crosstalk between the Wip1–mTORC1 axis and the Wip1–p53 axis in lifespan regulation at the organismal level will be important. Mice Wip1 −/− mice were backcrossed for at least five generations to C57BL/6 mice in our laboratory. p53 −/− and p21 −/− mice were C57BL/6 background. Wip1 −/− p53 −/− or Wip1 −/− p21 −/− double-knockout mice were generated by crossing Wip1 +/− mice with p53 +/− or p21 +/− mice. The recipient mice used for the competitive transplantation assays were either B6.SJL-PtprcaPep3b/Boy (CD45.1) mice or CD45.1/CD45.2 heterozygous mice (both were C57BL/6 background). The Animal Care and Ethics Committee at the Hangzhou Normal University approved all of the animal experiments in our study. Mice of both genders were used in the studies at age of 2–3 months (young mice) or 22–24 months (old mice). All mice were maintained in a pathogen-free environment and were fed a standard diet. Flow cytometry and cell sorting BM cells were incubated in a lineage cocktail containing antibodies against CD4 (1:100, RM4-5), CD8 (1:100, 53-6.7), Ter-119 (1:100, TER-119), CD11b (1:150, M1/70), Gr-1 (1:150, RB6-8C5) and B220 (1:100, RA3-6B2) for 30 min. After washing, the cells were incubated in CD34 (1:100, RAM34), CD48 (1:200, HM48-1), CD45.2 (1:100, 104), IL-7R (1:100, A7R34), Flt3 (1:100, A2F10), CD150 (1:100, TC15-12F12.2), CD45.1 (1:100, A20), Sca1 (1:100, E13-161.7), c-Kit (1:100, ACK2), CD16/32 (1:100, 93) and streptavidin. Side population cell analysis was performed using Hoechst 33342 (5 μg ml −1 , Sigma-Aldrich). All monoclonal antibodies were from BD Biosciences or eBioscience. For fluorescence detection of SA-β-gal activity, the cells were incubated in C 12 FDG (33 μM, Sigma-Aldrich) and a β-galactosidase substrate [50] . Before cell sorting, first, the BM cells were enriched with anti-antigen-presenting cell microbeads (Miltenyi Biotec) and then stained with antibodies for surface markers. Data acquisition and cell sorting were performed using a LSRII/Fortessa cell analyzer or an Influx cell sorter (BD Biosciences). The data were analysed using the FlowJo software. Transplantation assay For the BM transplantation assay, 1 × 10 6 BM cells from donor mice were injected into lethally irradiated recipient mice with or without competitor cells. For the second and third transplantations, 5 × 10 6 BM cells were serially transplanted into the next recipient mice. For HSC transplantation, 50 CD150 high -HSCs, 400 CD34 − LSK cells or 4,000 LSK cells were FACS-sorted, mixed with 1 × 10 6 or 5 × 10 5 competitor BM cells and transplanted into lethally irradiated mice. Colony-forming assay Fresh isolated 1 × 10 4 BM cells were cultured in methylcellulose semi-solid medium (M3434, Stemcell Technologies) for 14 days, and the numbers and sizes of the colonies were assessed via microscopy. For the single-cell colony-forming assay, the cells were individually sorted into 96-well plates and cultured for 14 days in liquid medium in the presence or absence of the p38 MAPK inhibitor SB203580 (5 μM) or the NF-κB inhibitor caffeic acid phenethyl ester (6 μg ml −1 ). Lentivirus production Lentivirus was produced in 293T cells after transfection of 12 mg p53-shRNA plasmid, 9 mg pspAX2 helper plasmid and 3 mg pMD2G.23. The virus was concentrated by centrifugation at 25,000 r.p.m. for 2.5 h at 4 °C, and the virus pellet was suspended in sterile PBS. p53-shRNA sequence: 5′-TGCTGTTGACAGTGAGCG cccactacaagtacatgtgtaatag TGAAGCCACAGATGTAT tacacatgtacttgtagtgga TGCCTACTGCCTCGGA-3′. 5-FU treatment The recipient mice were injected (intraperitoneally, i.p.) with (5 mg g −1 ) PIPC (InvivoGen) every other day for 4 days, followed by injections (i.p.) of (150 mg kg −1 ) 5-FU (Sigma) every week for 2 weeks. For cell cycle or apoptosis analysis, the mice were injected (i.p.) with (150 mg kg −1 ) 5-FU and were killed at the indicated time point. Analysis of the cell cycle and apoptosis Cell cycle analysis was performed via Ki67 and BrdU staining. For the long-term BrdU incorporation assay, BrdU (100 mg kg −1 ; BD Biosciences) was injected (i.p. ), followed by administration of (1 mg ml −1 ) BrdU in the drinking water for 10 days. BrdU incorporation was assessed via FACS analysis using a BrdU Flow Kit (BD Biosciences). Annexin V Apoptosis Detection Kits (eBioscience or BD Pharmingen) were used for the apoptosis analyses. For the in vitro assays, the cells were sorted and cultured in SFEM (Stemcell Technologies) medium containing (50 ng ml −1 ) SCF and (50 ng ml −1 ) TPO and were analysed via the BrdU incorporation and Annexin V staining assays. Blood cell counts PB from the postorbital vein was collected and analysed using a blood cell counter (Sysmex). Wip1 inhibitor and rapamycin treatment The mice were injected (i.p.) with the Wip1 inhibitor (CCT007093, 2.5 mg kg −1 in dimethylsulphoxide) every 12 h. Alternatively, BrdU (1 mg ml −1 ) and rapamycin (15 μg ml −1 ) were administered to the mice in the drinking water. The mice were killed 3 days after treatment, and the BM cells were collected for subsequent analysis. RNA purification and real-time PCR Total RNA was extracted from FACS-sorted cells using an RNeasy kit (Qiagen). qRT–PCR was performed using a CFX96 Real-Time System (Bio-Rad). The amount of target RNA was normalized to that of the endogenous control β-actin (Actb). The gene expression quantities were determined according to the relative C t method. Western blot analysis The cells were lysed in RIPA buffer and subjected to 15% SDS-PAGE followed by incubation with antibodies against PPM1D ( Wip1 ; 1:100, Santa Cruz), p53 (1:500, Cell Signaling), phosphorylated p53 (1:500, Cell Signaling), phosphorylated pS6K (1:1,000, Cell Signaling) and β-actin (1:5,000, Sigma). Ingenuity pathway analysis RNA was extracted using an RNeasy RNA extraction kit. Then, this RNA was amplified using a Qiagen amplification kit, fragmented and hybridized using the Mouse Expression Array 430 2.0 (Affymetrix). The microarray analysis was performed on the fold-change expression differences (HSCs), followed by IPA. Statistical analysis All data are expressed as the means±s.d. The statistical significance of the differences between the groups was calculated using an unpaired Student’s t -test, and the survival curve was analysed using a log-rank (Mantel-Cox) test. Accession codes: The microarray data sets have been deposited in the NCBI Gene Expression Omnibus (GEO) and are accessible at GEO accession number GSE58754. How to cite this article: Chen, Z. et al. Wip1 deficiency impairs haematopoietic stem cell function via p53 and mTORC1 pathways. Nat. Commun. 6:6808 doi: 10.1038/ncomms7808 (2015).